A synthetic biochemistry molecular purge valve module that maintains redox balance The greatest potential environmental benefit of metabolic engineering would be the production of high-volume commodity chemicals, such as biofuels. Yet, the high yields required for the economic viability of low-value chemicals is particularly hard to achieve in microbes owing to the myriad competing biochemical pathways. An alternative approach, which we call synthetic biochemistry, is to eliminate the organism by constructing biochemical pathways in vitro . Viable synthetic biochemistry, however, will require simple methods to replace the cellular circuitry that maintains cofactor balance. Here we design a simple purge valve module for maintaining NADP + /NADPH balance. We test the purge valve in the production of polyhydroxybutyryl bioplastic and isoprene—pathways where cofactor generation and utilization are unbalanced. We find that the regulatory system is highly robust to variations in cofactor levels and readily transportable. The molecular purge valve provides a step towards developing continuously operating, sustainable synthetic biochemistry systems. Metabolic engineering and synthetic biology have been employed for the production of high-value chemicals but has not been as successful in meeting the stringent economics of large-scale commodity chemical manufacturing [1] . Microbial systems are often hampered by a variety of technical challenges that make it hard to achieve cost competitiveness, including poor yields owing to competing pathways; low productivity caused by slow growth rates or difficulties in pathway optimization; contaminating microbial growth; product toxicity; and expensive product isolation [2] , [3] . Another approach that is beginning to receive attention is to perform complex biochemical transformations using mixtures of enzymes in a reaction vessel rather than within a cell. Building single, dedicated pathways in vitro can eliminate side reactions that occur in the cell, so that nearly 100% yields and fast reaction times are possible [3] , [4] , [5] . In vitro biochemical systems also allow for more precise control over optimization and product toxicity problems can be more easily diagnosed and mitigated [6] , [7] . Moreover, product extraction can be more facile. Traditionally, in vitro pathway construction has been relegated to use as a research tool or in applications that require only 1—3 enzymes for the production of chiral compounds and other high-value chemicals [1] , [8] , [9] . Improvements in protein expression and access to stable enzymes have made more complex systems possible, however [1] , [9] , [10] , [11] , [12] . In vitro biotransformation systems have been reported in recent years involving systems of over 30 enzymes [13] , [14] . One of the first modern studies in this area was an artificial pathway that produced hydrogen from starch [1] , [15] , [16] , [17] . The concept was recently advanced with a creative system that generated hydrogen from cellobiose at nearly 100% yields [16] . In another effort, hyper-thermophilic glycolysis enzymes were heterologously expressed, heat purified and assembled to convert glucose to n -butanol in 82% yield [18] . In another study, an elegantly simplified non-phosphorylative Entner–Doudoroff pathway from hyper-thermophilic archaea was constructed to produce ethanol and isobutanol in ~55% yields [19] . These pioneering studies illustrate the flexibility of synthetic biochemistry and the potential for high yields. A limiting feature of earlier work in synthetic biochemistry systems is the need to either feed the systems with high-energy cofactors, or if they are generated by the pathway in situ , balance their use to ensure regeneration. For example, in the Sieber pathway to generate ethanol and isopropanol from glucose [19] , the pathway was beautifully designed to reduce only 2 mol of NAD + to NADH during the catabolic phase and to reoxidize 2 mol of NADH in the anabolic phase. Thus, the utilization of NAD + was perfectly balanced allowing multiple passes through the pathway. In other systems, the pathways were also designed to maintain cofactor balance [18] . The requirement for perfect balance limits synthetic biochemistry in two ways, however. First, it places stringent constraints on pathway design, potentially limiting the types of chemicals that can be made. Second, it may ultimately limit the number of cycles the system can perform without adding additional, expensive high-energy cofactors. Why? If there is any spontaneous oxidation of NADH, it effectively creates an unintended cofactor imbalance because more NADH is required than would be expected based on the stoichiometry of the system. Thus, over time the levels of NADH will dissipate and the system will wind down. As the economic viability of a synthetic biochemistry system will likely depend on the ability to run the systems in a self-sustaining manner for long periods of time, we need to develop methods that can maintain high-energy cofactor levels without requiring perfect pathway stoichiometry. Ideally, we believe that a synthetic biochemistry system should be able to generate more high-energy cofactors in the catabolic phase of the pathway, than is needed in the anabolic phase of the pathway so that gradual losses by spontaneous ATP hydrolysis or NAD(P)H oxidation can be tolerated. On the other hand, if an excess of high-energy cofactors is produced, it is necessary to also find a way to dissipate excess production so that the reactions can proceed (that is, carbon flux can be maintained). In short, we need a way to maintain cofactor balance. If it were possible to regulate cofactor balance without affecting carbon flux, it would also allow for much more flexibility in pathway design. As a step towards this goal, we describe a synthetic biochemistry purge valve module to maintain the proper balance of NADPH and test whether this general approach can be applied for the production of the bioplastic polyhydroxybutyrate (PHB) and isoprene. PHB and other polyhydroxyalkanoates (PHAs) are biodegradable thermoplastics. PHAs can have characteristics similar to many popular petrochemical-derived polymers, but are nontoxic and biodegradable, so they are attracting increased attention as a possible green alternative to petroleum-based polymers in a wide range of applications [20] , [21] , [22] . The best characterized and most abundant PHA polymer is PHB that is naturally produced from acetyl-CoA as a carbon and energy storage mechanism in many organisms [22] . Currently, industrial production of PHB is done by in vivo batch culture processes under nutrient starvation. This process is typically very time consuming, requires large fermentation volumes and requires expensive methods for the extraction of PHB [20] . Prior attempts to produce bioplastic in vitro have required the addition of sacrificial substrates and a molar excess of cofactors to convert acetate to PHB [23] . Isoprene is a platform chemical for a variety of products, but it is mostly employed in the production of synthetic rubber [24] , [25] , [26] . The isoprenoid pathway also provides precursors for over 25,000 known biomolecules including drugs such as taxol and potential biofuels [27] . There have been a number of efforts to produce isoprene in microorganisms [24] , [26] , [28] , [29] and the best reported yield is 28% from glucose [24] . We recently showed that a synthetic biochemistry system could produce isoprene in >95% yield from pyruvate as long as high-energy cofactors were added [30] . Here we employ a purge valve system in a pathway to convert pyruvate into PHB that maintains sustainable reducing cofactor balance, without the requirement for perfect stoichiometric matching of cofactor generation and carbon usage. Further, we show that our purge valve module can be used as the basis for the production of other acetyl-CoA-derived products by applying it to the production of isoprene from pyruvate via the mevalonate pathway. Regulatory modules such as this can free us from having to perfectly balance cofactor utilization when designing synthetic biochemistry systems. Overview and design of pathway The biotransformation of pyruvate into PHB illustrates a basic cofactor imbalance problem that is encountered in biochemical systems. In particular, conversion of pyruvate to acetyl-CoA by pyruvate dehydrogenase (PDH) yields one molecule of NADH. However, the three-enzyme pathway (phaA, B and C) to PHB from acetyl-CoA utilizes only one half of a molecule of NADPH per acetyl-CoA. Thus, the canonical pathway produces an excess of reducing equivalents. Moreover, the reducing equivalents are of the wrong type (NADH rather than NADPH). We therefore designed a pathway, shown in Fig. 1a that can generate the correct cofactor and regulate its production. 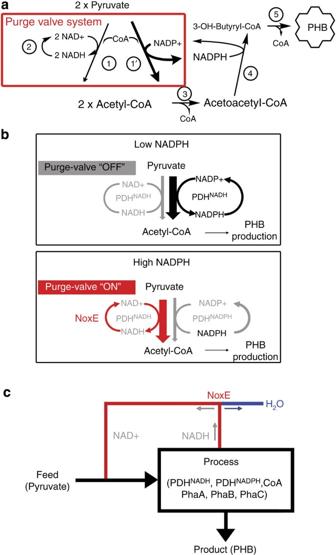Figure 1: A synthetic biochemistry purge valve system for the production of PHB. (a) Thein vitrometabolic pathway for the conversion of pyruvate to PHB. The pathway consists of six separate reactions: reaction 1 (PDHNADH), reaction 1′ (PDHNADPH), reaction 2 (NoxE), reaction 3 (PhaA), reaction 4 (PhaB) and reaction 5 (PhaC). The purge valve is highlighted in the red box. (b) How the purge valve is designed to function. At low NADPH (high NADP+), PDHNADPHreaction dominates, generating acetyl-CoA and NADPH from pyruvate and NADP+. The purge valve is effectively ‘off’. In high-NADPH (low NADP+) conditions, the PHDNADPHenzyme is starved for oxidized cofactor, shutting down this pathway to acetyl-CoA. In this situation, the PDHNADH/NoxE system takes over, producing only acetyl-CoA. In other words, the purge valve is effectively ‘on’. (c) A chemical engineering schematic of the purge valve system used in the production of PHB from pyruvate, involving a cofactor recycle loop. Figure 1: A synthetic biochemistry purge valve system for the production of PHB. ( a ) The in vitro metabolic pathway for the conversion of pyruvate to PHB. The pathway consists of six separate reactions: reaction 1 (PDH NADH ), reaction 1′ (PDH NADPH ), reaction 2 (NoxE), reaction 3 (PhaA), reaction 4 (PhaB) and reaction 5 (PhaC). The purge valve is highlighted in the red box. ( b ) How the purge valve is designed to function. At low NADPH (high NADP+), PDH NADPH reaction dominates, generating acetyl-CoA and NADPH from pyruvate and NADP + . The purge valve is effectively ‘off’. In high-NADPH (low NADP + ) conditions, the PHD NADPH enzyme is starved for oxidized cofactor, shutting down this pathway to acetyl-CoA. In this situation, the PDH NADH /NoxE system takes over, producing only acetyl-CoA. In other words, the purge valve is effectively ‘on’. ( c ) A chemical engineering schematic of the purge valve system used in the production of PHB from pyruvate, involving a cofactor recycle loop. Full size image In our design, we create a synthetic biochemistry ‘purge valve’ that effectively decouples the stoichometric production of NAD(P)H from acetyl-CoA ( Fig. 1 ). To this end, we employ a mixture of both an NAD + -utilizing wild-type (WT) PDH (PDH NADH ), a mutant PDH that utilizes NADP + (PDH NADPH ), and a water-generating NADH oxidase (NoxE) that specifically oxidizes NADH, but not NADPH [31] , [32] . By employing this metabolic node, we generate NADPH needed for PHB production from pyruvate, but also dissipate excess reducing equivalents in an autoregulatory manner. As illustrated in Fig. 1b , under low-NADPH, high-NADP + conditions, the mutant PDH NADPH can operate to generate acetyl-CoA and restore NADPH levels. Under high-NADPH, low-NADP + conditions, the PDH NADPH activity will automatically be choked off, and the WT PDH NADH will be used preferentially to produce acetyl-CoA and NADH. In this high-NADPH condition, the reducing equivalents are not needed. Because the reducing equivalents are produced in the form of NADH and not NADPH, they are eliminated by the oxidase, NoxE. The presence of NoxE ensures that NADH never builds up and the PDH NADH can always operate to generate carbon for the PHB pathway in the form of acetyl-CoA. The PDH NADH /PDH NADPH /NoxE system acts like a purge valve that opens under conditions of high NADPH to relieve the excess reducing equivalent ‘pressure’ (that is, buildup of NADH) and allow carbon flux to be maintained. An engineering schematic of the purge valve system is shown in Fig. 1c . Enzyme engineering and cofactor specificity To implement our purge valve module, we needed an NADP + -utilizing PDH. A mutant of Escherichia coli PDH has been engineered to have NADP + specificity by introducing mutations into the E3 enzyme (EcE3) [33] . The E. coli PDH proved too unstable for our system, however. We therefore engineered a mutant of the thermophilic Geobacillus stearothermophilus PDH that preferentially accepts NADP + with increased enzyme stability. Similar to the design of the E. coli PDH mutant, the G. stearothermophilus PDH mutant was designed by overlaying the known structure of the G. stearothermophilus E3 subunit (GsE3) [33] with the known structure of the related E. coli glutathione reductase, which utilizes NADP + (ref. 33 ) (REF or PDBID:1GET). The structural superposition allowed us to position the additional phosphate moiety in the active site of the GsE3, based on how it was placed in glutathione reductase (see Fig. 2 ). We could then design side-chain substitutions in GsE3 that might allow acceptance of the phosphate. We were guided by the prior successful design of the EcE3 enzyme, which shares 47% sequence identity with the GsE3 (refs 33 , 34 ). The mutations introduced into EcE3 were E206V, G207R, A208K, G209H and S213R (GsE3 numbering). After examining the changes in the context of the GsE3 structure, we decided to introduce all but G209H, because it appeared that the new His side chain might create steric clashes with nearby K224 and N237 residues. 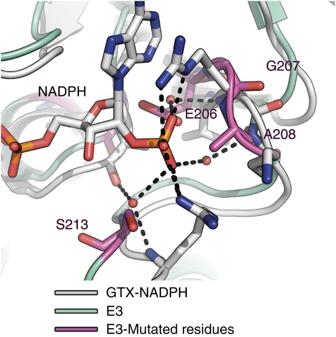Figure 2: Design of the PDHNADPHenzyme. The structures of the wild-typeG. stearothermophilusE3 subunit (E3, green backbone trace) is shown overlaid on the structure ofE. coliglutathione reductase (GTX-NADPH, grey backbone trace). The NADPH substrate from glutathione reductase is shown in stick representation, showing the placement of the phosphate moiety that needs to be accommodated. The residues changed to accept the phosphate (E206V, G207R, A208K and S213R) are shown in purple. Figure 2: Design of the PDH NADPH enzyme. The structures of the wild-type G. stearothermophilus E3 subunit (E3, green backbone trace) is shown overlaid on the structure of E. coli glutathione reductase (GTX-NADPH, grey backbone trace). The NADPH substrate from glutathione reductase is shown in stick representation, showing the placement of the phosphate moiety that needs to be accommodated. The residues changed to accept the phosphate (E206V, G207R, A208K and S213R) are shown in purple. Full size image The kinetic properties of the engineered and WT enzymes reveal that the mutations alter specificity as desired. The kinetic parameters are listed in Supplementary Table 1 . For the WT G. stearothermophilus enzyme (GsPDH NADH ), k cat is 11.2 times higher with NAD + than NADP + and k cat / K m is 1,150 times higher. For the engineered mutant (GsPDH NADPH ), k cat is 7.3 times higher with NADP + than NAD+ and k cat / K m is 21 times higher. Thus, we were able to flip the specificity of the PDH enzyme. The GsPDH NADH and GsPDH NADPH enzymes (henceforth designated PDH NADH and PDH NADPH ) were much more stable than their E. coli counterparts. As shown in Supplementary Fig. 1 , the G stearothermophilus enzymes retained ~50% activity after 1 h incubation at 67 °C, whereas the E. coli PDH enzymes were completely inactivated at 50 °C. A second key requirement of the purge valve design is the use of an NADH oxidase with high cofactor specificity. We chose NoxE from Lactococcus lactis as it is a water-forming NADH oxidase so it does not generate any toxic products such as hydrogen peroxide [31] , [32] , [35] . As shown in Table 1 , the K cat of NoxE is 248.8 times greater with NADH than NADPH and k cat / K m is 9,900 times greater. Table 1 Enzymes used in this work. Full size table Enzyme catalysed production of PHB from pyruvate The enzymes chosen for use in this work are listed in Table 1 . In the initial tests, we only employed the WT, PDH NADH complex and NoxE to generate acetyl-CoA and supplied NADPH exogenously. After optimizing enzyme ratios in this simple system, we then added the mutant PDH NADPH to test in situ generation of NADPH. Finally, the amount of PDH NADPH was optimized, keeping the other enzymes fixed. The progress of the optimized pyruvate to PHB reaction is shown in Fig. 3 along with a control lacking the last enzyme, phaC. Both reactions had a PDH NADPH :PDH NADH ratio of 40:1. At this ratio, the NADPH levels rise rapidly (A 340 ) and are maintained throughout the time course (NoxE rapidly oxidizes NADH so changes in A 340 reflect only changes in NADPH levels). At the same time, PHB granules are produced as monitored by A 600 (ref. 36 ). 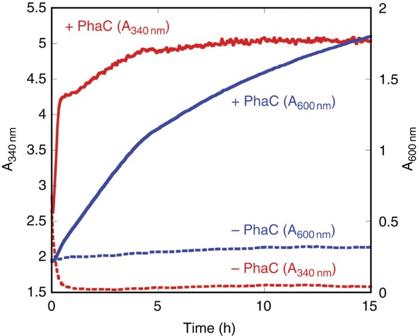Figure 3: Production of PHB using an optimized system. In this reaction, the production of PHB is monitored by an increase A600(blue) caused by precipitation of the PHB granules. No increase is seen in the absence of the PHB polymerase, PhaC. The production of PHB is confirmed by a gas chromatography assay (see text). The A340(red) monitors the level of NADPH because no NADH is allowed to build up because of the presence of NoxE. The purge valve system maintains a high level of NADPH throughout the reaction. Figure 3: Production of PHB using an optimized system. In this reaction, the production of PHB is monitored by an increase A 600 (blue) caused by precipitation of the PHB granules. No increase is seen in the absence of the PHB polymerase, PhaC. The production of PHB is confirmed by a gas chromatography assay (see text). The A 340 (red) monitors the level of NADPH because no NADH is allowed to build up because of the presence of NoxE. The purge valve system maintains a high level of NADPH throughout the reaction. Full size image We assayed the PHB production using a gas chromatography method and found that the optimized reaction produced 2.45±0.5 mg ml −1 of PHB from 50 mM pyruvate, which represents nearly complete conversion (94±20%) of pyruvate to plastic. In the optimized system, we started with 0.5 mM NADP + , so achieving 94% yield requires over 90 turnovers of the NADP + cofactor, indicating a high level of system sustainability. The stability of the full system was assessed by mixing components together and then initiating the reaction at various time delays. The decrease in extent of the reaction is shown in Supplementary Fig. 2 . We find that the extent of reaction remains ~50% after 2 days. Autoregulatory behaviour of purge valve The regulatory behaviour of the purge valve is better seen at sub-optimal enzyme concentrations and ratios of PDH NADPH to PDH NADH that slow down the response time. In the optimized assay (40:1 mol ratio of PDH NADPH :PDH NADH ), we observed a rapid rise in NADPH levels, which was sustained throughout. In the non-optimal systems shown in Fig. 4 , the purge valve cannot respond as rapidly to drops in NADPH concentrations so we can observe variations in NADPH levels as the system develops. We still observe a rapid initial rise in NADPH levels, but as intermediates build up, the consumption starts to outstrip NADPH production. Eventually, the system compensates by generating higher levels of NADPH. The restoration of NADPH levels would be impossible without the proper operation of the purge valve system. 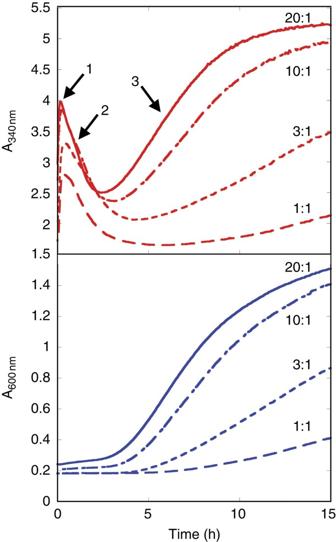Figure 4:Time course of pyruvate to PHB optimization reaction using sub-optimal ratios of PDHNADPHand PDHNADH. The A340traces (red), monitoring NADPH levels fall into three distinct phases. A fast initial reduction of NADPH by the PDHNADPHis followed by a slow oxidation of NADPH by PhaB as the intermediate levels rise. As the reaction proceeds, the purge valve effectively turns off and NADPH levels rise again. The evolution of the system coincides with the increase at A600(blue), which represents the precipitation of the PHB granules from solution. Figure 4: Time course of pyruvate to PHB optimization reaction using sub-optimal ratios of PDH NADPH and PDH NADH . The A 340 traces (red), monitoring NADPH levels fall into three distinct phases. A fast initial reduction of NADPH by the PDH NADPH is followed by a slow oxidation of NADPH by PhaB as the intermediate levels rise. As the reaction proceeds, the purge valve effectively turns off and NADPH levels rise again. The evolution of the system coincides with the increase at A 600 (blue), which represents the precipitation of the PHB granules from solution. Full size image The system is robust to cofactor levels To test whether the system was robust to changes in cofactor levels, we varied the initial cofactor concentrations in the reactions and measured the yields of PHB. Each reaction was constructed with combinations of NAD + , NADH, NADP + or NADPH at either 0.1 or 1 mM and the production of PHB was monitored by the final OD at 600 nm. All of the reaction conditions were compared with the optimized reaction that produced nearly complete conversion of pyruvate to PHB and, as shown in Fig. 5 , were within random variation (see also Supplementary Table 3 ). This result indicates that the purge valve can compensate readily for changes in cofactor concentrations and reduction states. 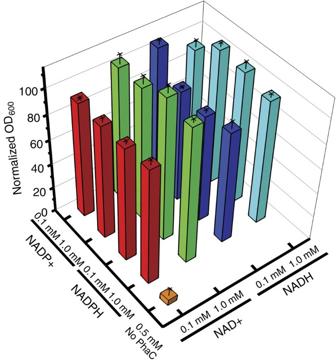Figure 5: The purge valve system is robust. The graph shows relative yield of PHB upon starting with different amounts of each of the cofactors. The relative yields represent the ratio of the final A600for the reaction, relative to the final A600for the optimized reaction. All reactions show a relatively robust yield in comparison with the negative control lacking the final phaC enzyme (orange bar). The error bars reflect the s.d. of three independent reactions. The data are listed inSupplementary Table 3. Figure 5: The purge valve system is robust. The graph shows relative yield of PHB upon starting with different amounts of each of the cofactors. The relative yields represent the ratio of the final A 600 for the reaction, relative to the final A 600 for the optimized reaction. All reactions show a relatively robust yield in comparison with the negative control lacking the final phaC enzyme (orange bar). The error bars reflect the s.d. of three independent reactions. The data are listed in Supplementary Table 3 . Full size image Porting the purge valve system to isoprene production To test the versatility of the molecular purge valve and whether it can be applied as a general platform for the production of a diverse array of acetyl-CoA-derived compounds, we used the PDH purge valve to produce isoprene via the acetyl-CoA-dependent mevalonate pathway. We have previously described the in vitro production of isoprene from pyruvate, which required the use of exogenously added NADPH [30] . Similar to the PHB pathway, the mevalonate pathway has an inherently different carbon and cofactor stoichiometry. In particular, the mevalonate pathway requires three acetyl-CoA and two NADPH for the production of isoprene (see Fig. 6a ). Thus, system sustainability requires generation and regulation of NADPH levels. 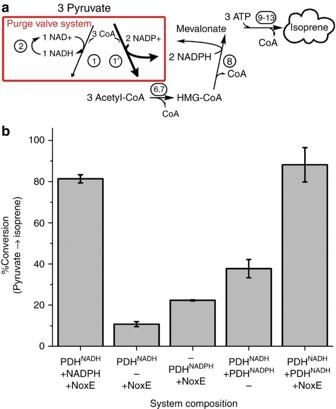Figure 6: Employing the purge valve for the production of isoprene. (a) Thein vitrometabolic pathway for the conversion of pyruvate to isoprene. The purge valve highlighted in the red box consists of the same enzymes/reactions as inFig. 1. In the mevalonate pathway, three acetyl-CoA are used to make HMG-CoA (enzymes 6 and 7). HMG-CoA is reduced by HMGR (enzyme 8) with two NADPH to give mevalonate. Three ATP are then used to convert mevalonate to isopentenyl pyrophosphate followed by production of isoprene (enzymes 9–13). (b) The graph shows the dependence of isoprene production on the purge valve. No purge valve was used in the first reaction (PDHNADH, NADPH and NoxE). NADPH was simply added and NADH recycled using NoxE. The final experiment (PDHNADH, PDHNADPHand NoxE) shows results employing the full purge valve system. Leaving out any component of the purge valve system resulted in marked decreases in isoprene production. Each reaction was performed in duplicate and the error was calculated as the s.d. of the two replicates. Figure 6: Employing the purge valve for the production of isoprene. ( a ) The in vitro metabolic pathway for the conversion of pyruvate to isoprene. The purge valve highlighted in the red box consists of the same enzymes/reactions as in Fig. 1 . In the mevalonate pathway, three acetyl-CoA are used to make HMG-CoA (enzymes 6 and 7). HMG-CoA is reduced by HMGR (enzyme 8) with two NADPH to give mevalonate. Three ATP are then used to convert mevalonate to isopentenyl pyrophosphate followed by production of isoprene (enzymes 9–13). ( b ) The graph shows the dependence of isoprene production on the purge valve. No purge valve was used in the first reaction (PDH NADH , NADPH and NoxE). NADPH was simply added and NADH recycled using NoxE. The final experiment (PDH NADH , PDH NADPH and NoxE) shows results employing the full purge valve system. Leaving out any component of the purge valve system resulted in marked decreases in isoprene production. Each reaction was performed in duplicate and the error was calculated as the s.d. of the two replicates. Full size image We tested whether the purge valve system can replace exogenously added NADPH in the production of isoprene. As shown in Fig. 6b , the full purge valve system produces an 88.2±8.4% yield from 3 mM pyruvate. This yield is even higher than the 81.4±2.0% yield obtained if we add NADPH exogenously ( Fig. 6b ). If we leave out any of the purge valve components (PDH NADPH , PDH NADH or NoxE), yields are markedly reduced. Thus, the purge valve system is clearly transportable to other synthetic biochemistry systems. Maintaining proper cofactor balance is an essential part of generating flux and providing a driving force through an enzymatic pathway. In vivo , the enzymatic specificity for the cofactors NADH and NADPH are typically used to control the carbon flux through catabolic and anabolic pathways, respectively. Organisms typically sense the reduction state of these cofactors and use this information to upregulate or downregulate catabolic and anabolic pathways to cope with environmental changes. In vitro systems, however, do not have the myriad peripheral pathways that facilitate this fine control. Moreover, the natural anabolic and catabolic specificities for NADH and NADPH complicate in vitro biotransformations. Synthetic biochemistry systems have often dealt with these problems by careful considerations of cofactor stoichiometry in pathway design, through the use of expensive sacrificial metabolites, re-engineering enzymes so that only a single cofactor type is needed, adding excess cofactors, or constantly adding intermediates to the reaction mix to sustain the process. In this work, we created a robust node of control to balance the production and consumption of NADPH and NADH in a self-regulating and self-balancing manner. To our knowledge, this is the first in vitro pathway that maintains cofactor balance without requiring adherence to stoichiometry in the generation and utilization of cofactors to ensure carbon flux. In part because the system can sustain high levels of NADPH, we can drive the transformation to near completion, converting pyruvate to either PHB or isoprene at nearly 100% of the theoretical yield. Moreover, the high yields in our system are robust to 10-fold variations in cofactor levels. Ultimately it will be necessary to expand this pathway to incorporate the conversion of low-cost substrates such as glucose or other sugars into pyruvate, which would involve the glycolysis pathway or parts of the glycolysis pathway. Indeed a synthetic biochemistry system employing glycolysis has been demonstrated previously [5] . Building more complex compounds from acetyl-CoA such as fatty acids, polyketides and other isoprenoids will also require the incorporation and recycling of ATP. Thus, it would be desirable to develop simple methods to regulate the ATP/ADP levels within the context of synthetic biochemistry. ATP regulation will be an interesting challenge for future synthetic biochemistry pathway designs. Ultimately, developing regulatory systems similar to the purge valve employed here will free synthetic biochemistry system design from having to consume the high-energy cofactors during the anabolic phase in perfect stoichiometric balance. Thus, our approach can help diversify the chemical targets of synthetic biochemistry. Materials Miller Luria-Bertani (LB) media or Miller LB-agar (BD Difco) was used for growth of bacterial strains in liquid or solid media. E. coli BL21-Gold(DE3) (B, F-, ompT, hsdS B, (r B −,m B −), dcm+,Tet r , gal λ, (DE3) endA Hte ) (Agilent) was used as a host for both cloning and expression of recombinant proteins using pET vectors. E. coli TOP10(DE3) (F- mcrA Δ(mrr-hsdRMS-mcrBC) φ80lacZΔM15 ΔlacX74 nupG recA1 araD139 Δ(ara-leu)7697 galE15 galK16 rpsL(Str R ) endA1 λ − ) was used for expression of recombinant proteins from the pBAD/p15A vector [37] . Plasmids pET28a(+) and pET22b(+) were purchased from Novagen. HotStart Taq Mastermix (Denville) was used for gene amplification from genomic or plasmid DNA. Phusion DNA polymerase (Finnizymes), Taq DNA ligase (MCLab), and T5 Exonuclease (Epicenter) were purchased separately and used to make the assembly master mix (AMM) used for cloning (ref). ATP, (±)-α-lipoic acid, pyruvate, coenzyme A and NAD + were from Sigma. Plasmid construction The expression plasmids for the PHB enzymes were constructed from the pET28a plasmid backbone using the Nde1- and Sac1-cut sites to produce constructs with an N-terminal 6 × His tag for purification. The genes encoding acetyl-CoA acetyltraferase (phaA; YP_725941) and acetoacetyl-CoA reductase (phaB; YP_725942) [23] were amplified and cloned from Ralstonia eutropha genomic DNA. The gene encoding PHB synthase [38] , [39] (phaC; HE_610111) was synthesized and codon optimized for expression in an E. coli host at Life Technologies before being subcloned into the pET28a expression vector. For the isoprene pathway, the constructs were the same as described in reference [30] . E. coli BL21-Gold cells were used as the host strain for enzyme expression. All enzymes were expressed in LB media supplemented with 50 μg ml −1 kanamycin and were induced with 0.2 mM isopropyl-β- D -1-thiogalactopyranoside added to the culture at the end of log phase growth. The phaA, phaB, MVK, PMVK and IspS were induced at 37 °C overnight and phaB, THL/HMGR, HMGS and IDI were induced at 18 °C overnight. The phaC was induced at 25 °C for 5 h before harvesting. Enzyme purification Cells from 0.5 l of culture were harvested by centrifugation and resuspended in 150 mM Tris pH 7.5, 100 mM NaCl. The cells were lysed on ice with sonication and the cell debris was removed by 12,000 g centrifugation at 4 °C. The supernatant was then mixed with 5 ml nickel-nitrilotriacetic acid agarose and after 30 min, the agarose slurry was loaded onto a gravity column and washed with five-column volumes of 100 mM Tris pH 7.5, 100 mM NaCl and 15 mM imidazole. The enzyme was then eluted with 250 mM imidazole, 100 mM Tris pH 7.5. The resulting enzyme was dialysed into 50 mM Tris pH 7.5, 50 mM NaCl and stored at 4 °C. Expression vectors for PDH subunits and E. coli LplA The E1, E2 and E3 domains were all amplified separately from G. stearothermophilus genomic DNA (ATCC) using primers that contained 15–20 bp complementary to the gene and 15–20 bp complementary to the multiple cloning site in the vector where the gene would be placed. The genes encoding E1α and E1β were amplified together from G. stearothermophilus genomic DNA and cloned into pET28a(+) that had been digested with Nco I and Xho I. This created a tagless construct for E1 expression under control of the T7 promoter where E1α translation uses the ribosomal binding site from the pET28 vector while E1β uses the endogenous ribosomal binding site from G. stearothermophilus. The E2 and E3 domains were amplified separately and cloned into pET22b(+) digested with Nde I and Xho I or pET28a(+) digested with Nco I and Xho I, respectively, to create tagless E2 and E3 constructs. The E. coli lipoate protein ligase, LplA, was amplified from E. coli K12 genomic DNA and assembled into pBAD/p15A [37] digested with Xho I and Eco RI to create 6 × His-LplA. Overexpression and purification of PDH subunits and LplA All E. coli strains were grown at 37 °C in LB-media supplemented with appropriate antibiotic (100 μg ml −1 ampicillin, 50 μg ml −1 kanamycin or 34 μg ml −1 chloramphenicol). For all constructs, 5 ml of overnight starter culture was used to inoculate 1 l of LB-media. Once the OD 600 reached 0.6, 0.3 mM IPTG (pET vectors) or 0.02% arabinose (pBAD/p15A) was added to induce protein expression. After 16 h, cells were harvested, resuspended (4 ml g −1 wet cells) in 50 mM Tris-Cl pH 7.5, 0.1 M NaCl (buffer A), lysed by sonication and cell debris removed by centrifugation at 30,000 g for 20 min. E. coli lysate (25 ml) containing 6 × His-LplA was loaded onto a 3-ml nickel-nitrilotriacetic acid resin (Qiagen), washed with 25 ml buffer A containing 10 mM imidazole and eluted with 5 ml buffer A containing 250 mM imidazole. Pure 6 × His-LplA was then stored at 4 °C until use. The individual domains of G. stearothermophilus PDH were partially purified from E. coli lysates by heat before modification and reconstitution of the PDH complex. E1αβ-, E2- or E3-containing lysates were incubated at 65 °C for 35 min to heat denature E. coli proteins followed by centrifugation at 30,000 g for 20 min to pellet the precipitated proteins. Nearly all of the PDH domains remain in the supernatant. Next, the E2 domain was lipoated in the heated extract by the addition of 1 mM (±)-α-lipoic acid, 2 mM ATP, 3 mM MgCl 2 and 50 μg of purified 6 × His-LplA. The lipoation reaction was then allowed to proceed with gentle mixing overnight at 25 °C, yielding lipoated E2 (E2lip). After lipoation, E1αβ, E2lip and E3 were mixed in a 3:1:3 molar ratio and incubated for at least 1 h at 25 °C to form the active GsPDH complex. The GsPDH complex was then isolated by ultracentrifugation (Beckman) for 4 h at 95,000 g . The resulting yellow pellet was resuspended in 20 mM Tris-Cl, pH 7.5 in 1/50 the starting volume and assayed for activity [33] , [34] , [40] . SDS–polyacrylamide gel electrophoresis analysis confirmed the presence of all four domains and indicated that the preparation was >90% pure. The reconstituted complex was stored at 4 °C until use. Enzyme activity and optimization NoxE was assayed by monitoring the oxidation of NAD(P)H at 340 nm. The assay was carried out in 100 mM Tris–HCl pH 7.5, 5 mM MgCl 2 , 5 mM KCl and 0.2 mM NAD(P)H. WT and mutant PDH were assayed by monitoring the reduction of NAD(P) + at 340 nm. The assay was carried out in 50 mM Tris pH 7.5, 5 mM MgCl 2 , 5 mM pyruvate, 1 mM CoA and 0.5 mM of NAD(P) + . PhaC was assayed by monitoring the absorbance of the hydrolysis of the thioester bond of the substrate 3HBCoA at 235 nm. The assay was carried out in 100 mM Tris pH 7.5, 5 mM MgCl 2 and 0.15 mM 3HBCoA. Activity of NADPH-consuming isoprene pathway enzymes were monitored with the decrease of absorbance at 340 nm. Activity of ATP-consuming enzymes were monitored with a coupled assay system with pyruvate kinase and lactate dehydrogenase at 340 nm. The amount of each enzyme in the reconstituted isoprene pathway described below is show in Supplementary Table 2 . Final PHB reaction conditions and analysis The optimized self-sustaining reaction for the biotransformation of pyruvate to PHB was composed of 250 mM Tris pH 7.5, 5 mM MgCl, 5 mM KCl, 0.5 mM CoA, 0.1 mM NAD + , 0.5 mM NADP + , 50 mM pyruvate, 2 μg PDH NADH , 76 μg PDH NADPH , 23 μg phaA, 14 μgphaB and 32 μg phaC in a final reaction volume of 200 μl. The reactions were initiated with the addition of pyruvate, which was left out of the initial mixture. All PHB reactions were performed at room temperature. For testing the autoregulatory behaviour of the purge valve, some enzyme concentrations were sub-optimal: 5 μg phaA, 2.5 μg phaB and 1.9 μg phaC. To assay for PHB, the reactions were lyophilized and incubated with 1 ml chloroform, 0.45 ml methanol and 0.05 ml H 2 SO 4 to hydrolyse the polymer and generate methyl 3-hydroxybutyrate. The reactions were extracted with 0.5 ml water and 1 μl of the chloroform layer was applied to a 0.25-micron HP-Innowax column using a HP 5890 Series II gas chromatogram. The gas chromatography method used an injection temperature that was held at 35 °C for 5 min before it was increased to 275 °C over 40 min. The peak intensities were compared with an authentic standard to assess concentrations. Isoprene reaction conditions and analysis In vitro production of isoprene was performed as described previously [30] with the following changes. 200 μl reactions were set up in 2-ml gas-tight vials containing enzymes, 3 mM pyruvate, 15 mM ATP, 0.6 mM CoA, 0.2 mM NAD+, 0.4 mM NADP+ (or 5 mM NADPH), 10 mM MgCl 2 , 20 mM KCl and 0.1 mM thiamine pyrophosphate in 100 mM Tris-Cl pH 8.5 and incubated at 32 °C for 18 h. Isoprene production was monitored by direct sampling of 100 μl of the headspace using a 100-μl gas-tight syringe. The headspace was analysed by GC-FID (HP5980II) equipped with a GS-GasPro column (0.32 mm × 30 m, Agilent) as described previously [30] . The carrier gas was helium with a flow rate of 5 ml min −1 . The oven temperature was kept at 120 °C for 3 min then raised to 230 °C at 5 C min −1 then to 250 °C at 20 °C min −1 and held for at 250 °C for 9 min. The inlet and detector temperatures were kept at 270 and 330 °C, respectively. The amount of isoprene produced was quantified by comparison with a standard curve of various isoprene concentrations sampled in the same manner. How to cite this article: Opgenorth, P. H. et al . A synthetic biochemistry molecular purge valve module that maintains redox balance. Nat. Commun. 5:4113 doi: 10.1038/ncomms5113 (2014).